Distinct loops in arrestin differentially regulate ligand binding within the GPCR opsin G-protein-coupled receptors are universally regulated by arrestin binding. Here we show that rod arrestin induces uptake of the agonist all- trans -retinol in only half the population of phosphorylated opsin in the native membrane. Agonist uptake blocks subsequent entry of the inverse agonist 11- cis -retinal (that is, regeneration of rhodopsin), but regeneration is not blocked in the other half of aporeceptors. Environmentally sensitive fluorophores attached to arrestin reported that conformational changes in loop V−VI (N-domain) are coupled to the entry of agonist, while loop XVIII−XIX (C-domain) engages the aporeceptor even before agonist is added. The data are most consistent with a model in which each domain of arrestin engages its own aporeceptor, and the different binding preferences of the domains lead to asymmetric ligand binding by the aporeceptors. Such a mechanism would protect the rod cell in bright light by concurrently sequestering toxic all- trans -retinol and allowing regeneration with 11- cis -retinal. Despite the variety of different ligands bound by G-protein-coupled receptors (GPCR), this large family of cell surface receptors shares a common seven transmembrane helical structure and activation mechanism. Receptor activation involves both an outward tilt of helix 6 and an extension of helix 5, which opens a deep cleft within the cytoplasmic face of the receptor [1] , [2] , [3] , [4] , [5] . This opening enables binding of the helical C-terminus of the alpha subunit of the G-protein [2] , [5] , a heterotrimeric protein that carries the signal into the cell interior. GPCR signalling is regulated by a small family of structurally conserved arrestin proteins [6] . In the case of rhodopsin, phosphorylation of the receptor C-tail following activation enables arrestin to bind and thus block G-protein activation. For other GPCRs, arrestin binding can additionally lead to receptor endocytosis and G-protein-independent signalling [7] . The GPCR rhodopsin mediates the first steps of visual signal transduction in the rod cell [8] , [9] . In the inactive state, the inverse agonist 11- cis -retinal is linked by a protonated Schiff base to the receptor. Absorption of light isomerises the retinal ligand to the agonist all- trans -retinal (ATR), which results in the active Meta II species [3] . Meta II is unstable and decays to the aporeceptor opsin upon hydrolysis of the retinal Schiff base and release of ATR. In the native membrane environment, the re-entry of ATR into opsin does not occur, whereas 11- cis -retinal can readily enter opsin and thereby regenerate rhodopsin [10] . Rhodopsin has traditionally been considered an exception among GPCRs, as its agonist comes not from the surroundings but is created by light directly within the binding pocket. Thus we were surprised in this study to discover that, in the presence of arrestin, exogenous ATR entered the binding pocket of phosphorylated opsin (OpsP) and reformed the retinal Schiff base. Intriguingly, agonist entered only half of receptors. We probed the structural basis of this observation using site-directed fluorescence spectroscopy, and we identified two loops on either domain of arrestin that have different binding preferences with respect to receptor activation state. The differentiation of arrestin's two domains allows arrestin to adopt different modes of binding for the different functional forms of receptor, and this adaptability in receptor binding is well suited to its specialized role in the visual system as well as its ubiquitous regulation of GPCRs. ATR stimulates arrestin binding to OpsP ATR has long been known to stimulate arrestin binding to OpsP [11] , but no study has undertaken a quantitative characterisation of this interaction. We determined the affinity, stoichiometry and salt sensitivity of arrestin binding to OpsP, with or without ATR, and in comparison to phosphorylated Meta II (Meta II-P). Arrestin binding was measured by a centri-fugal pull-down assay using the N , N ′-dimethyl- N -(iodoacetyl)- N ′-(7-nitrobenz-2-oxa-1,3-diazol-4-yl)ethylenediamine (NBD)-labelled arrestin mutant A366C (A366NBD) [12] , and we confirmed that every phosphorylated receptor in our preparation was capable of binding arrestin in the light-activated form ( Fig. 1 ). When all receptors in the native rod outer segment (ROS) membrane were light-activated, one arrestin bound for every 1.4 Meta II-P ( Fig. 2a ; Supplementary Table S1 ). This stoichiometry implies a mixture of 1:1 and 1:2 binding and differs from what we recently reported [12] owing to an improvement in sample preparation that yielded higher levels of receptor phosphorylation ( Supplementary Methods ). Although it is established that arrestin binds Meta II-P with a low nanomolar K d [13] , [14] , [15] , similar to what we measured by Meta II-stabilization at 2 °C ( Fig. 1 ), we measured a higher apparent K d of ~300 nM at 22 °C due to influence of Meta II decay [12] and other experimental limitations (Methods). In contrast to Meta II-P, arrestin bound to OpsP with lower affinity (apparent K d =1.5 μM), and this interaction was easily disturbed by salt ( Supplementary Fig. S1 and Supplementary Table S1 ), indicating that arrestin-bound OpsP primarily electrostatically ( Supplementary Note 1 ). The addition of ATR to OpsP resulted in an arrestin-binding stoichiometry and apparent affinity very similar to that for Meta II-P ( Fig. 2a ) and likewise introduced salt-resistant hydrophobic-binding elements. Notably, arrestin binding to OpsP/ATR was more salt sensitive than arrestin binding to Meta II-P ( Supplementary Fig. S1 and Supplementary Table S1 ). 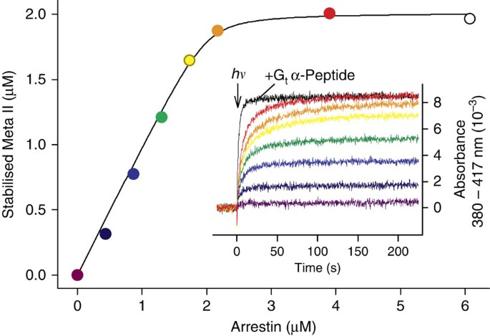Figure 1: Functional test of receptor phosphorylation. Arrestin was titrated against 10 μM RhoP (pH 8, 2 °C), and the amount of stabilized Meta II following an activating flash (20%) was measured as shown in the inset. A fit of equation (3) to the data indicated that one arrestin bound for every light-activated RhoP with an apparentKdof 27 nM, which corresponds to a trueKdof 2.2 nM when corrected for the Meta I/Meta II equilibrium12,13,59. Inset—binding to and stabilisation of Meta II over its precursor Meta I results in an increase in absorbance (380–417 nm). In the control experiment (black trace), 300 μM Gtα-peptide (the high-affinity analogue peptide derived from the C-terminus of the α-subunit of transducin, VLEDLKSCGLF) stabilized 100% of receptors as Meta II60. The coloured traces correspond to the arrestin titration. Experiments were carried out as described previously12. Figure 1: Functional test of receptor phosphorylation. Arrestin was titrated against 10 μM RhoP (pH 8, 2 °C), and the amount of stabilized Meta II following an activating flash (20%) was measured as shown in the inset. A fit of equation (3) to the data indicated that one arrestin bound for every light-activated RhoP with an apparent K d of 27 nM, which corresponds to a true K d of 2.2 nM when corrected for the Meta I/Meta II equilibrium [12] , [13] , [59] . Inset—binding to and stabilisation of Meta II over its precursor Meta I results in an increase in absorbance (380–417 nm). In the control experiment (black trace), 300 μM G t α-peptide (the high-affinity analogue peptide derived from the C-terminus of the α-subunit of transducin, VLEDLKSCGLF) stabilized 100% of receptors as Meta II [60] . The coloured traces correspond to the arrestin titration. Experiments were carried out as described previously [12] . 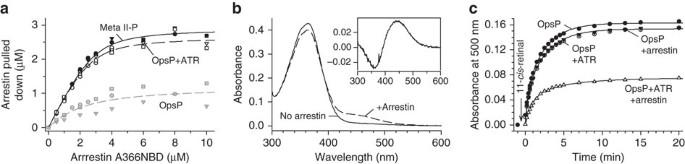Figure 2: Arrestin reforms Meta II-P from OpsP and ATR. (a) Arrestin was titrated against 4 μM light-induced Meta II-P (black symbols), 4 μM OpsP+40 μM ATR (white symbols) or 4 μM OpsP (grey symbols) in isotonic buffer, and arrestin binding was measured by pull down. Curves were fit as described in the Methods, and apparentKdand stoichiometry values are listed inSupplementary Table S1. (b) OpsP (4 μM) and ATR (4 μM) were mixed together with or without arrestin (4 μM) in 50 mM HEPES buffer pH 7 without salt. After equilibration, 20 mMt-bHA was added to remove peripheral Schiff bases, followed by acid denaturation and detergent solubilisation. The resulting absorbance spectra of the samples are shown. Inset—difference spectrum calculated by subtracting the spectrum without arrestin from that with arrestin. (c) The time course of regeneration of OpsP (4 μM) by 11-cis-retinal (20 μM) was followed by monitoring the absorbance at 500 nm (arrestin: 4 μM; ATR: 40 μM; 50 mM HEPES buffer pH 7 without salt, 20 °C). Full size image Figure 2: Arrestin reforms Meta II-P from OpsP and ATR. ( a ) Arrestin was titrated against 4 μM light-induced Meta II-P (black symbols), 4 μM OpsP+40 μM ATR (white symbols) or 4 μM OpsP (grey symbols) in isotonic buffer, and arrestin binding was measured by pull down. Curves were fit as described in the Methods, and apparent K d and stoichiometry values are listed in Supplementary Table S1 . ( b ) OpsP (4 μM) and ATR (4 μM) were mixed together with or without arrestin (4 μM) in 50 mM HEPES buffer pH 7 without salt. After equilibration, 20 mM t -bHA was added to remove peripheral Schiff bases, followed by acid denaturation and detergent solubilisation. The resulting absorbance spectra of the samples are shown. Inset—difference spectrum calculated by subtracting the spectrum without arrestin from that with arrestin. ( c ) The time course of regeneration of OpsP (4 μM) by 11- cis -retinal (20 μM) was followed by monitoring the absorbance at 500 nm (arrestin: 4 μM; ATR: 40 μM; 50 mM HEPES buffer pH 7 without salt, 20 °C). Full size image ATR is Schiff base linked in the ternary complex We next explored how ATR was bound in complex with OpsP and arrestin. In dark-state rhodopsin and light-activated Meta II, the retinal ligand is attached through a Schiff base linkage to Lys-296 of opsin. Besides the main retinal-binding pocket of opsin, secondary retinal-binding sites may exist where retinal binds non-covalently and partially activates the receptor [10] . We probed whether ATR was Schiff base linked in complex with OpsP and arrestin using acidification, which denatures protein and traps the retinal Schiff base in a protonated form that absorbs maximally at 440 nm. Nonspecific retinal Schiff bases, which readily form between ATR and the solvent-exposed amines present in phospholipids and proteins, were removed before acidification with o-tert -butyl-hydroxylamine ( t -bHA). T -bHA cannot access the retina-binding pocket in Meta II [16] . With this experimental strategy, we observed that arrestin allowed the formation of t -bHA-resistant retinal Schiff base in mixtures of OpsP and ATR ( Fig. 2b ). A difference spectrum showed that arrestin shifted a portion of ATR from free (360 nm) to Schiff base-linked (440 nm; Fig. 2b , inset). We used this experimental approach to later quantify arrestin-dependent retinal Schiff base formation. Arrestin-dependent ATR uptake blocks regeneration We next assessed the influence of ATR and arrestin on the uptake of 11- cis -retinal by OpsP to reform rhodopsin (that is, regeneration). In the absence of any ATR or arrestin, regeneration was complete after 20 min at 20 °C ( Fig. 2c ). In the presence of an excess of either ATR or arrestin, regeneration proceeded with similar kinetics, and ~5% of OpsP was not regenerated. In contrast, the presence of both ATR and arrestin caused 55% of OpsP not to be regenerated within the time course of the experiment. The remaining 45% of OpsP regenerated with kinetics similar to that of OpsP alone. As 11- cis -retinal entry was blocked, we can infer that ATR likely resided within the retinal-binding pocket [10] . Based on this result, and in combination with the evidence for t -bHA-resistant retinal Schiff base ( Fig. 2b ), we conclude that arrestin binding leads to the formation of a reversible form of Meta II-P [4] from OpsP and exogenous ATR. Binding stoichiometry We next determined the stoichiometries and apparent affinities for the arrestin/OpsP/ATR complex by titrating either ATR or arrestin. We used the three basic assays described above. Arrestin binding was measured by pull down, and ATR binding was measured by both acid trapping of retinal Schiff base as well as blockage of regeneration ( Fig. 3a,b ). K d and stoichiometry values were determined by fitting appropriate equations to the data (Methods). Overall, the data indicated that ATR bound the complex with an apparent K d of 3–5 μM ( Table 1 ). This K d value is apparent, as it describes the association of arrestin, ATR and OpsP in coupled equilibria. Furthermore, all experiments indicated that at most one molecule of ATR could bind for every two receptors, even in the presence of a great excess of ATR and arrestin. The data also indicated an overall arrestin to receptor-binding ratio between 1:1 and 1:2 in the presence of saturating ATR. This observed binding ratio can be interpreted as a mixture of agonist-dependent and -independent (that is, mediated by electrostatic interactions with phosphates) binding. The stoichiometry of the agonist-dependent interaction is seen in the ATR titration, where arrestin binding was measured by pull down ( Fig. 3a , red trace). In the absence of ATR, 0.8 μM arrestin was bound electrostatically to OpsP, causing the titration curve to be shifted on the y axis. ATR induced an additional 2 μM arrestin to bind to 4 μM receptor. Thus, we conclude a functional stoichiometry two OpsP receptors, one ATR, and one arrestin. Furthermore, formation of the complex requires both receptors to be sufficiently phosphorylated, as OpsP preparations with lower phosphorylation level yielded correspondingly lower levels of arrestin and ATR binding ( Fig. 3c,d ). However, in the case of light-induced Meta II-P, the lower receptor phosphorylation level resulted in an arrestin-receptor-binding ratio of 1:2 ( Fig. 3d ). These results suggest that OpsP/ATR and light-induced Meta II-P have different phosphorylation requirements with respect to arrestin binding ( Supplementary Note 2 ). 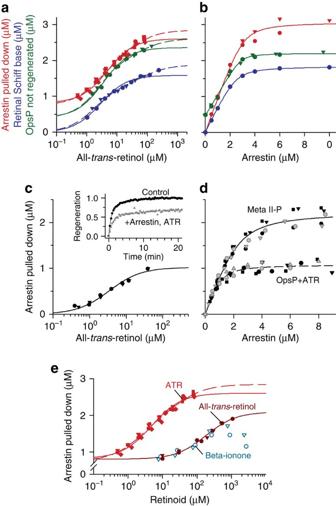Figure 3: Arrestin and retinoid titrations. (a) ATR was titrated against 4 μM arrestin+4 μM OpsP. (b) Arrestin was titrated against 4 μM OpsP+40 μM ATR. Arrestin binding (red), retinal Schiff base formation (blue) and blocked rhodopsin regeneration (green) were measured as described in the text. All experiments were performed in HEPES buffer pH 7 without salt, except for the pull-down experiment in (a) (red), where isotonic buffer was necessary to reduce agonist-independent arrestin binding. For the regeneration data (green), the fitted curves intercept theyaxis at ~0.5, reflecting the fact that not all OpsP was regenerated due to experimental constraints (Methods). Both single-site (solid traces) and two-site (dashed traces) binding models were fit to the retinal titration data. (c) ATR was titrated against 4 μM arrestin+4 μM OpsP using an OpsP preparation in which ~70% of receptors were able to bind arrestin as light-induced Meta II-P. The fitted curve reports an apparentKdof 3.4 μM and a stoichiometry of one arrestin per 4 receptors. Inset—time course of regeneration of OpsP (4 μM) with 11-cis-retinal (20 μM) in the absence or presence of arrestin (4 μM) and ATR (40 μM). (d) Arrestin titrations using mutants A366NBD (black symbols) or S344NBD (grey symbols) were performed against 4 μM Meta II-P or 4 μM OpsP+40 μM ATR using the same under-phosphorylated receptors as in (c). The fitted curves report that that one arrestin bound for every 1.8 Meta II-P or 3.6 μM OpsP/ATR (200 nM<Kd<300 nM). For both (c) and (d), arrestin binding in isotonic buffer was measured by pull down. (e) ATR and beta-ionone were titrated against 4 μM arrestin+4 μM OpsP (100% phosphorylated) in isotonic buffer, and arrestin binding was measured by pull down. The ATR data and fits from panel (a) are shown for reference. Note that beta-ionone caused scattering artefacts at higher concentrations. For all panels, data points from independent experiments are represented by differently shaped symbols, and the combined data points were used to fit the binding curves described in the Methods. Figure 3: Arrestin and retinoid titrations. ( a ) ATR was titrated against 4 μM arrestin+4 μM OpsP. ( b ) Arrestin was titrated against 4 μM OpsP+40 μM ATR. Arrestin binding (red), retinal Schiff base formation (blue) and blocked rhodopsin regeneration (green) were measured as described in the text. All experiments were performed in HEPES buffer pH 7 without salt, except for the pull-down experiment in ( a ) (red), where isotonic buffer was necessary to reduce agonist-independent arrestin binding. For the regeneration data (green), the fitted curves intercept the y axis at ~0.5, reflecting the fact that not all OpsP was regenerated due to experimental constraints (Methods). Both single-site (solid traces) and two-site (dashed traces) binding models were fit to the retinal titration data. ( c ) ATR was titrated against 4 μM arrestin+4 μM OpsP using an OpsP preparation in which ~70% of receptors were able to bind arrestin as light-induced Meta II-P. The fitted curve reports an apparent K d of 3.4 μM and a stoichiometry of one arrestin per 4 receptors. Inset—time course of regeneration of OpsP (4 μM) with 11- cis -retinal (20 μM) in the absence or presence of arrestin (4 μM) and ATR (40 μM). ( d ) Arrestin titrations using mutants A366NBD (black symbols) or S344NBD (grey symbols) were performed against 4 μM Meta II-P or 4 μM OpsP+40 μM ATR using the same under-phosphorylated receptors as in ( c ). The fitted curves report that that one arrestin bound for every 1.8 Meta II-P or 3.6 μM OpsP/ATR (200 nM< K d <300 nM). For both ( c ) and ( d ), arrestin binding in isotonic buffer was measured by pull down. ( e ) ATR and beta-ionone were titrated against 4 μM arrestin+4 μM OpsP (100% phosphorylated) in isotonic buffer, and arrestin binding was measured by pull down. The ATR data and fits from panel ( a ) are shown for reference. Note that beta-ionone caused scattering artefacts at higher concentrations. For all panels, data points from independent experiments are represented by differently shaped symbols, and the combined data points were used to fit the binding curves described in the Methods. Full size image Table 1 Summary of binding parameters for the arrestin/OpsP/ATR complex. Full size table Incidentally, both ATR and beta-ionone also induced arrestin binding to OpsP with an apparent K d ~40 times higher than that for ATR ( Fig. 3e ). These results indicate that, while ATR forms a Schiff base when it enters the ligand-binding pocket of arrestin-bound OpsP, the Schiff base is not mandatory to induce arrestin binding to OpsP. Arrestin traps half of ATR after Meta II-P decay The experiments presented above were all carried out at low micromolar concentration, as necessitated by the measurement techniques and so that meaningful titration analyses could be carried out. Under these conditions, an excess of exogenous ATR was required to achieve full association, as the apparent K d of ATR for the complex is 3–5 μM. In the rod cell, levels of ATR are potentially high but would never exceed opsin concentration, except perhaps in disease states caused by mutations in vital retinal-clearing enzymes like all- trans -retinol dehydrogenase (RDH) and the ABCA4 transporter [17] . To better emulate the physiologically relevant situation, we monitored retinal Schiff base within more concentrated, fully regenerated ROS membranes ( Fig. 4a ). In these experiments, ATR was not added exogenously but was instead released as Meta II-P decayed. Under physiological conditions, half of ATR was trapped in the binding pocket long after Meta II decay was complete. In the absence of arrestin, only ~10% of retinal Schiff base remained after Meta II decay was complete, which likely represented Meta III, a side product of Meta II decay [18] . As arrestin induced trapping of half the ATR at both 30 and 300 μM rhodopsin concentration, we presume this phenomenon occurs at the 3-mM rhodopsin concentration found in the rod cell [19] . 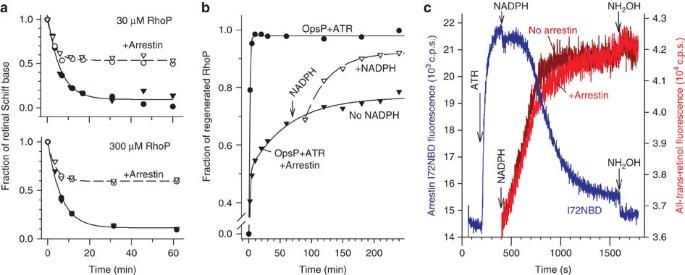Figure 4: Physiological context of ATR trapping. (a) Isolated ROS membranes containing 30 μM RhoP (upper panel) or 300 μM RhoP (lower panel) were fully photoactivated without arrestin (closed symbols) or with arrestin (open symbols), which was present at the physiologically relevant ratio of 0.67 arrestin per rhodopsin42,43. Meta II-P decay was monitored as the decrease int-bHA-resistant retinal Schiff base. Each experiment was performed twice in isotonic buffer at 37 °C. (b) A sample containing 4 μM OpsP+20 μM ATR, with (triangles) or without (circles) 4 μM arrestin was monitored for regeneration after the addition of 11-cis-retinal (12 μM). NADPH (200 μM), the essential cofactor of RDH, was added 60 min after the start of regeneration to an arrestin-containing sample (open triangles). Experiments were performed in 50 mM HEPES buffer pH 7 without salt, 20 °C. (c) The fluorescence of arrestin I72NBD (2 μM, blue trace) in the presence of OpsP (2 μM) was monitored over time after subsequent additions of ATR (4 μM,t=200 s), NADPH (200 μM,t=400 s) and NH2OH (10 mM,t=1600 s). ATR formation after addition of NADPH to samples of OpsP (2 μM) and ATR (4 μM) was monitored in the absence (dark red) or presence of 2 μM unlabelled arrestin (red). Experiments were performed in 50 mM HEPES buffer pH 7 without salt, 35 °C. Figure 4: Physiological context of ATR trapping. ( a ) Isolated ROS membranes containing 30 μM RhoP (upper panel) or 300 μM RhoP (lower panel) were fully photoactivated without arrestin (closed symbols) or with arrestin (open symbols), which was present at the physiologically relevant ratio of 0.67 arrestin per rhodopsin [42] , [43] . Meta II-P decay was monitored as the decrease in t -bHA-resistant retinal Schiff base. Each experiment was performed twice in isotonic buffer at 37 °C. ( b ) A sample containing 4 μM OpsP+20 μM ATR, with (triangles) or without (circles) 4 μM arrestin was monitored for regeneration after the addition of 11- cis -retinal (12 μM). NADPH (200 μM), the essential cofactor of RDH, was added 60 min after the start of regeneration to an arrestin-containing sample (open triangles). Experiments were performed in 50 mM HEPES buffer pH 7 without salt, 20 °C. ( c ) The fluorescence of arrestin I72NBD (2 μM, blue trace) in the presence of OpsP (2 μM) was monitored over time after subsequent additions of ATR (4 μM, t =200 s), NADPH (200 μM, t =400 s) and NH 2 OH (10 mM, t =1600 s). ATR formation after addition of NADPH to samples of OpsP (2 μM) and ATR (4 μM) was monitored in the absence (dark red) or presence of 2 μM unlabelled arrestin (red). Experiments were performed in 50 mM HEPES buffer pH 7 without salt, 35 °C. Full size image RDH activity dissociates the complex To further put our results into physiological context, we explored the influence of RDH activity on the ability of arrestin to block regeneration in complex with OpsP and ATR. RDH reduces toxic ATR to nontoxic all- trans -retinol in the rod cell and requires nicotinamide adenine dinucleotide phosphate oxidase (NADPH) as a cofactor [20] . RDH is present in isolated ROS membranes, and its enzymatic activity is preserved even after extensive receptor phosphorylation [11] . In the absence of RDH activity, OpsP regenerated quickly in the presence of an excess of ATR ( Fig. 4b ), but only ~50% of OpsP regenerated after 10 min in the presence of both ATR and arrestin. Over the next several hours, ~25% more OpsP was regenerated. This slow regeneration reflects the fact that arrestin-bound Meta II-P exists in equilibrium with its dissociated components, and 11- cis -retinal can diffuse into the binding pocket of OpsP while the complex is transiently dissociated. This process was quite slow, as ATR was in excess to 11- cis -retinal. In contrast, regeneration was greatly accelerated by the addition of NADPH. By reducing free ATR to all- trans -retinol, RDH activity removed the block of regeneration. We next directly observed the link between RDH activity and conformational changes in arrestin using the fluorescently labelled arrestin mutant I72NBD ( Fig. 4c ). The spectral properties of arrestin mutants labelled at site 72 with solvent-sensitive fluorophores have been correlated to activating conformational changes in arrestin that occur upon binding Meta II-P [21] , [22] , [23] . We observed that the fluorescence of I72NBD in the presence of OpsP increased upon addition of ATR. Upon the subsequent addition of NADPH, I72NBD fluorescence decreased in a sigmoidal manner. At the same time, all- trans -retinol fluorescence increased, indicating that the agonist-induced conformational changes in arrestin reversed as ATR was reduced. The kinetics of all- trans -retinol formation and the reversal of conformational changes in arrestin did not match in the initial phase because RDH first reduced the excess free ATR. As the concentration of free ATR decreased, so did the probability that the complex would reform, and the concentration of the complex slowly decreased. Distinct binding preferences of two arrestin loops Multiple studies have localised the receptor-binding interface to both concave surfaces of the arrestin molecule [24] . We individually mutated multiple sites within the binding interface to cysteine and attached the environmentally sensitive fluorophore NBD ( Fig. 5a ). The fluorescence of NBD is enhanced in nonpolar, hydrophobic environments. Of all the sites tested, only probes on or near loop V−VI (residues 68–78, hereafter referred to as loop-72) or loop XVIII−XIX (residues 336–344, hereafter referred to as loop-344) showed large changes when arrestin bound to Meta II-P ( Fig. 5b ). These results are consistent with studies that have identified loop-72 (refs [21] , [22] , [23] , [24] , [25] , [26] ) and loop-344 (refs [12] , [21] , [25] ) as being important in receptor binding. 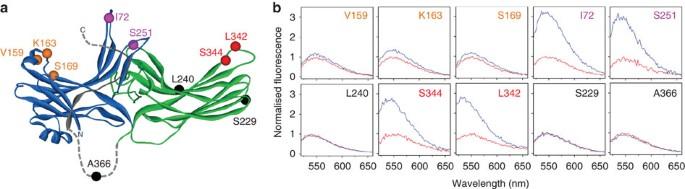Figure 5: Site-directed fluorescence experiments. (a) Location of single cysteine substitutions and attachment of the NBD fluorophore on a model of arrestin derived from the crystal structure (PDB code 1CF1). The N-domain is coloured blue, the C-domain is green and the C-terminus is grey. (b) For each panel, 1 μM fluorescently labelled arrestin was mixed with a fourfold excess of dark-state RhoP. Emission spectra were recorded before (red traces) and after (blue traces) a 10-s illumination (>495 nm). Spectra were background-subtracted and normalised. Figure 5: Site-directed fluorescence experiments. ( a ) Location of single cysteine substitutions and attachment of the NBD fluorophore on a model of arrestin derived from the crystal structure (PDB code 1CF1). The N-domain is coloured blue, the C-domain is green and the C-terminus is grey. ( b ) For each panel, 1 μM fluorescently labelled arrestin was mixed with a fourfold excess of dark-state RhoP. Emission spectra were recorded before (red traces) and after (blue traces) a 10-s illumination (>495 nm). Spectra were background-subtracted and normalised. Full size image We next compared how these two loops are involved in arrestin binding to different receptor species: dark-state phosphorylated rhodopsin (RhoP), light-induced Meta II-P and OpsP in the absence or presence of an excess of ATR. We measured the fluorescence of the labelled arrestin mutants in the presence of increasing concentrations of receptor, and the actual amount of arrestin binding was measured in parallel by pull down ( Fig. 6 ). Note that salt was excluded from these experiments to maximise binding. Hence, higher arrestin affinity for all receptor species was observed ( Supplementary Fig. S2 ) as compared with experiments performed in isotonic buffer ( Fig. 2a ). For both I72NBD and S344NBD, dark-state RhoP elicited no change in fluorescence, although pull-down experiments showed that arrestin binding occurred ( Fig. 6a,e ), and bimane probes placed at these sites showed a decrease in solvent accessibility when arrestin-bound dark-state RhoP ( Supplementary Fig. S3 and Supplementary Note 3 ). Arrestin I72NBD bound to dark-state RhoP with significantly higher affinity than arrestin S344NBD. We hypothesise that the NBD probe at site 72 destabilises the basal conformation of arrestin [23] and exposes buried phosphate-binding elements in arrestin [24] , thereby increasing its affinity for phosphorylated receptor. In the case of light-activated Meta II-P, the fluorescence changes of both labelled arrestin mutants mirrored the actual amount of arrestin binding, with a binding ratio between 1:1 and 1:2 ( Fig. 6b,f ). With regard to OpsP binding, the fluorescence changes of arrestin S344NBD mirrored the actual amount of arrestin binding with a stoichiometry of one arrestin per two receptors ( Fig. 6g ). Note that the higher fluorescence intensity of arrestin S344NBD in the presence of saturating OpsP as compared with Meta II-P was likely due to the lack of quenching species derived from the retinal chromophore. In contrast to arrestin S344NBD, the fluorescence and pull-down results for arrestin I72NBD did not mirror one another ( Fig. 6c ). Arrestin I72NBD bound to OpsP with an affinity and stoichiometry similar to that for Meta II-P, yet the fluorescence of I72NBD was minimally affected by OpsP. When ATR was added to OpsP, the binding ratio reported by pull down was between 1:1 and 1:2 for both mutants ( Fig. 6d,h ). Although arrestin binding was directly reflected in fluorescence changes of the NBD probe at site 344, the fluorescence of the probe at site 72 saturated at an arrestin-receptor ratio of 1:2. As the increase in I72NBD fluorescence was directly proportional to the amount of ATR that entered OpsP, and this fluorescence change was reversed upon reduction of ATR to ATR ( Fig. 4c ), we conclude that conformational changes of loop-72 are directly linked to the presence of agonist in the binding pocket of the receptor. In contrast, S344NBD generally reported the amount of arrestin physically bound to the membrane surface, except in the case of dark-state RhoP. Hence, the role of loop-344 in receptor binding is independent of the activation state of the receptor. 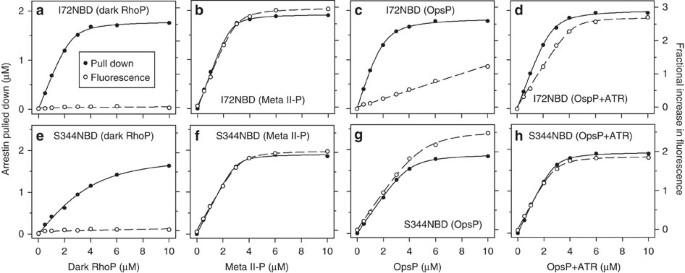Figure 6: Receptor titrations. (a) Dark-state RhoP was titrated against 2 μM arrestin I72NBD. (b) Light-induced Meta II-P was titrated against 2 μM arrestin I72NBD. (c) OpsP was titrated against 2 μM arrestin I72NBD. (d) OpsP plus a 10-fold molar excess of ATR was titrated against 2 μM arrestin I72NBD. (e) Dark-state RhoP was titrated against 2 μM arrestin S344NBD. (f) Light-induced Meta II-P was titrated against 2 μM arrestin S344NBD. (g) OpsP was titrated against 2 μM arrestin S344NBD. (h) OpsP plus a 10-fold molar excess of ATR was titrated against 2 μM arrestin S344NBD. Arrestin binding was measured by pull down (closed symbols), and the steady-state fluorescence was measured in parallel on identical samples (open symbols). In the case of the OpsP/ATR titrations, 20 mMt-bHA was added before fluorescence measurements to remove nonspecific retinal Schiff bases. The fluorescence is expressed as the fractional increase over that of unbound arrestin. For each panel, the left axis refers to arrestin pulled down, and the right axis refers to fluorescence. Each point represents the average of two independent experiments, which were performed in 50 mM HEPES buffer pH 7. Figure 6: Receptor titrations. ( a ) Dark-state RhoP was titrated against 2 μM arrestin I72NBD. ( b ) Light-induced Meta II-P was titrated against 2 μM arrestin I72NBD. ( c ) OpsP was titrated against 2 μM arrestin I72NBD. ( d ) OpsP plus a 10-fold molar excess of ATR was titrated against 2 μM arrestin I72NBD. ( e ) Dark-state RhoP was titrated against 2 μM arrestin S344NBD. ( f ) Light-induced Meta II-P was titrated against 2 μM arrestin S344NBD. ( g ) OpsP was titrated against 2 μM arrestin S344NBD. ( h ) OpsP plus a 10-fold molar excess of ATR was titrated against 2 μM arrestin S344NBD. Arrestin binding was measured by pull down (closed symbols), and the steady-state fluorescence was measured in parallel on identical samples (open symbols). In the case of the OpsP/ATR titrations, 20 mM t -bHA was added before fluorescence measurements to remove nonspecific retinal Schiff bases. The fluorescence is expressed as the fractional increase over that of unbound arrestin. For each panel, the left axis refers to arrestin pulled down, and the right axis refers to fluorescence. Each point represents the average of two independent experiments, which were performed in 50 mM HEPES buffer pH 7. Full size image The salient finding of this study on the visual receptor opsin ( Fig. 7a,b ) and rod arrestin (arrestin-1) ( Fig. 7c,d ) is that the differentiated binding preferences of the two domains of arrestin allows arrestin to accommodate the different functional forms of RhoP. Arrestin binding to dark-state RhoP is primarily electrostatic in nature [27] . Although residues in both domains in arrestin have been implicated in binding to dark-state RhoP [25] , [28] , our fluorescence results suggest that neither loop-72 nor loop-344 is deeply embedded in hydrophobic protein or membrane interfaces. Upon light-activation of RhoP, both loops are buried in hydrophobic environments. As the observed stoichiometry lay between the expected values for 1:1 and 1:2 binding, we conclude that arrestin can bind one or two Meta II-P molecules. We propose a binding model in which loop-72 tightly engages the activated receptor in a phosphorylation-dependent way [22] , [25] ( Fig. 7e ), consistent with the co-localization of loop-72 and the arrestin-activating phosphate-sensing elements in the N-domain [24] . In contrast, loop-344 engages either the membrane or a neighbouring receptor, regardless of the phosphorylation status of this second receptor. This assignment is consistent with the implication of the C-domain in phosphorylation-independent, low-affinity arrestin binding to Meta II [28] . Furthermore, the lack of a phosphorylation requirement for loop-344 engagement of neighbouring Meta II explains why we previously observed 1:2 binding in samples with lower receptor phosphorylation level [12] . 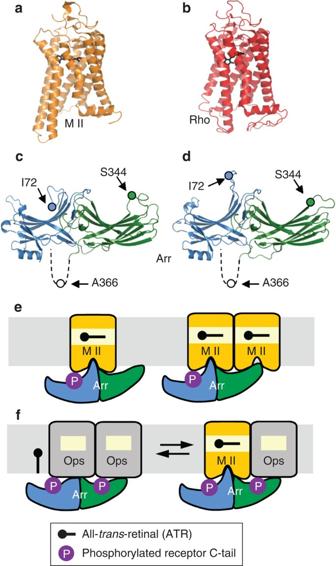Figure 7: Model of different binding modes of arrestin. (a) Crystal structure of Meta II (M II) (PDB code 3PXO). (b) Rhodopsin (Rho) (1U19), which is similar to inactive opsin in conformation30. (c) Arrestin with closed conformation of loop-72 (molecule D from 1CF1). (d) Arrestin with extended conformation of loop-72 (molecule A from 1CF1). The N-domain is coloured blue, the C-domain is coloured green and the C-terminus has been omitted for clarity. Sites labelled in this study are indicated. (e) As described in the text, arrestin binds light-induced Meta II-P in 1:1 or 1:2 complexes. (f) Arrestin binds functional dimers of OpsP, in which agonist (ATR) can enter one protomer and thereby reform Meta II-P. Meta II-P decay results in an equilibrium of free and bound ATR. Figure 7: Model of different binding modes of arrestin. ( a ) Crystal structure of Meta II (M II) (PDB code 3PXO). ( b ) Rhodopsin (Rho) (1U19), which is similar to inactive opsin in conformation [30] . ( c ) Arrestin with closed conformation of loop-72 (molecule D from 1CF1). ( d ) Arrestin with extended conformation of loop-72 (molecule A from 1CF1). The N-domain is coloured blue, the C-domain is coloured green and the C-terminus has been omitted for clarity. Sites labelled in this study are indicated. ( e ) As described in the text, arrestin binds light-induced Meta II-P in 1:1 or 1:2 complexes. ( f ) Arrestin binds functional dimers of OpsP, in which agonist (ATR) can enter one protomer and thereby reform Meta II-P. Meta II-P decay results in an equilibrium of free and bound ATR. Full size image Arrestin-bound Meta II-P ultimately decays to OpsP and free ATR [11] , [22] . A key finding of this study is that arrestin facilitates the uptake of ATR by OpsP. Re-entry of ATR likely requires the active conformation of opsin [29] . In native membranes and in the absence of arrestin, ATR cannot re-enter the binding pocket ( Supplementary Fig. S4 ), presumably because the conformational equilibrium of opsin is heavily shifted in favour of inactive receptor [30] . We postulate that it is loop-72 of arrestin that facilitates agonist re-entry by shifting the conformational equilibrium of OpsP. The entry of ATR and the engagement of loop-72 then mutually stabilise one another in the high-affinity arrestin/Meta II-P complex. This interpretation is consistent with the observed coupling of agonist uptake and conformational changes in arrestin loop-72. Furthermore, a peptide representing this loop stabilises Meta II with millimolar affinity and adopts a helical conformation when bound to Meta II [26] . It is tempting to speculate that, similar to the C-terminus of the alpha subunit of G-protein, loop-72 of arrestin inserts into the cleft that opens on the cytoplasmic face of the active receptor [2] , [5] . In contrast, loop-344 of arrestin apparently does not facilitate agonist uptake, as this loop is engaged by inactive or active receptor and therefore does not affect the conformational equilibrium of OpsP. The fact that only half the OpsP population can take up ATR implies that arrestin can access only half the receptor population in such a way that agonist uptake is facilitated. Given the differences between loop-72 and loop-344, the simplest and therefore most likely explanation for the asymmetry of agonist uptake is that a single arrestin binds two OpsP molecules ( Fig. 7f ). The OpsP molecule bound by the N-domain of arrestin can take up ATR with a concomitant extension of loop-72 (ref. 23 ), and the OpsP molecule bound by the C-domain is engaged by loop-344, but this interaction does not lead to agonist uptake. The receptor bound by loop-344 is free to take up 11- cis -retinal, and this event does not appear to disrupt the complex, consistent with dark-state rhodopsin being similar to inactive opsin in its conformation [30] . Considering our finding that arrestin requires two OpsP molecules to stimulate agonist uptake in one OpsP, phosphate-sensing elements in both domains of arrestin are implied. Although no evidence currently exists for a C-domain phosphate sensor, no study, as far as we are aware, has specifically targeted arrestin residues used in OpsP binding. Notably, multiple solvent-exposed basic residues are clustered within the concave face of the C-domain that could potentially bind the phosphorylated receptor C-tail [31] . In brief, the two receptors in the arrestin-bound OpsP/ATR complex function as an asymmetric dimer [32] with regard to arrestin-dependent agonist uptake. As we cannot presently conclude whether the two co-organized receptors are necessarily in direct physical interaction, we use the term functional dimer. Given that pull-down analysis reported a ratio between 1:1 and 1:2 for arrestin binding to both light-induced Meta II-P and OpsP/ATR, one could conclude that arrestin also forms 1:1 or 1:2 complexes with OpsP, and some other unknown mechanism besides functional dimers determines which half of receptors can take up agonist. However, despite their similarities in arrestin-binding stoichiometry, light-induced Meta II-P and OpsP/ATR are markedly different with respect to their salt sensitivity and the stoichiometry reported by the agonist-sensitive conformational changes of loop-72 on arrestin. These differences likely originate from the different ways the two active receptor species are generated (that is, by light or by the interaction of arrestin with OpsP) and reflect the different binding modes arrestin adopts with light-induced Meta II-P and OpsP/ATR ( Fig. 7e,f ). From a physiological point of view, the different binding modes of arrestin correspond well to the functional needs of the cell at different light intensities. In the single photon range, arrestin binds monomeric Meta II-P to quench signalling. As the lighting level increases and photoactivates more rhodopsin, arrestin also binds dimeric Meta II, only one protomer of which need be phosphorylated. As the average receptor phosphorylation level increases in continuous bright light [33] , the rod cell switches from photoreceptor to survival mode [24] , [34] , in which ATR is sequestered in complex with arrestin-bound OpsP. The benefit of such a mechanism is clear given the toxicity of ATR and the association of its by-products with disease [35] , [36] , [37] , [38] . As rhodopsin is present at a cellular concentration of 3 mM [19] , and every photoactivation event results in the release of a molecule of ATR, normal daytime lighting levels present a real challenge to rod cell survival. Physiological conditions seem poised to allow for arrestin-dependent sequestration of ATR, as continuous bright light leads to both highly phosphorylated opsin [33] , [39] , [40] and the translocation of arrestin to the ROS [41] , [42] (resulting in an arrestin to receptor ratio between 1:1 and 1:2 (refs [42] , [43] )). Importantly, this sequestration does not block the reduction of ATR by RDH ( Fig. 4b,c ), consistent with the fact that ATR is released from the complex as Meta II-P decays, and RDH binds ATR with at least threefold higher affinity than arrestin-bound OpsP [20] . Arrestin-bound OpsP would serve as a sink for ATR that cannot immediately be reduced by RDH and would be vital during those times when the rate of photoactivation outpaces ATR reduction [44] or when NADPH is limited [45] . During continuous light exposure, rhodopsin regeneration is supported by delivery of 11- cis -retinal from neighbouring pigment epithelium cells [19] . Our results show that each arrestin-bound receptor pair can simultaneously act as a sink for ATR and 11- cis -retinal, which would both protect the rod cell and support continual regeneration. In summary, arrestin serves not only to quench Meta II signalling, but also protects the rod cell in bright light. This idea is consistent with the fact that rod arrestin knockout mice suffer retinal degeneration [46] that is likely due to excessive signalling through the G-protein pathway in dim light but is signalling-independent in bright light [47] . Within the wider family of GPCRs, the binding of β-arrestin increases the apparent affinity of the receptor for agonist [48] , [49] , [50] , [51] , [52] . Hence, β-arrestin binding stabilizes the agonist-binding receptor conformation, just as we have shown for visual arrestin. Given our findings, we expect that the N-domain of β-arrestin stabilizes the active receptor conformation, whereas the C-domain less specifically engages neighbouring receptor or membrane. The asymmetric ability of arrestin to stimulate ligand binding within receptor dimers may explain why β-arrestin was observed to induce high-affinity ligand binding in only a fraction (~30 to 60%) of membrane-bound β2-adrenergic receptors [48] . In another study, about half of ligand bound to phosphorylated N -formyl-peptide receptor was observed to have an extremely slow off-rate in the presence of arrestin [49] . Besides quenching GPCR signalling, β-arrestins also mediate receptor internalisation in clathrin-coated pits. There are splice variants of β-arrestin that differ in the loop analogous to loop-344 in rod arrestin [53] , and the longer splice variant has been observed to engage clathrin by means of this hydrophobic loop [54] . Considering that some ligands stimulate receptor internalisation while others do not, different ligand-binding modes that differentially engage the C-domain of arrestin is an intriguing possibility. Furthermore, many GPCR dimers are known to bind ligand asymmetrically [32] , and our results point to a role for arrestin in this process. In summary, the bilobed nature of arrestin is key to its versatility. The N-domain of arrestin mediates binding to agonist-activated receptor, whereas the less specific C-domain may serve various functions depending on the requirements of the biological system. Reagent preparation ROS membranes were isolated from frozen bovine retina (W.L. Lawson Company, USA) using a modified form of the widely used method of Papermaster [55] . Opsin was phosphorylated using the native rhodopsin kinase [56] , and membranes were subsequently washed with buffer to remove associated ROS proteins. A detailed protocol regarding the preparation of OpsP is included as Supplementary Methods . Recombinant bovine arrestin mutants lacking native cysteine and tryptophan residues (C63A, C128S, C143A and W194F) were expressed and purified exactly as described previously [57] . Single-cysteine substitution mutants were labelled with the cysteine-reactive fluorophore NBD (Molecular Probes, Invitrogen) as described [12] . ATR (Sigma-Aldrich) was used to generate 11- cis -retinal by light exposure, and both isoforms were subsequently purified using high pressure liquid chromatography [58] . All- trans -retinol and beta-ionone were purchased from Sigma-Aldrich and used without further purification. Centrifugal pull-down assay Binding of NBD-labelled arrestin mutants to ROS membranes was measured essentially as described previously [12] . In this study, a lower centrifugal force (16,000 g ) was found to be sufficient to pellet the membranes, as the minimal washing steps used in our current preparation yielded ROS membranes that were larger and more intact. In addition, we found that it was important to perform the centrifugation at room temperature, as binding of arrestin to OpsP was highly affected by temperature. Quantification of retinal Schiff base Samples containing OpsP, ATR and arrestin (100 μl) were incubated in the dark at room temperature for at least 30 min. Nonspecific peripheral Schiff bases were first removed with addition of 20 mM t -bHA [16] . After 2 min, 5 μl of 4N HCl was added to denature the proteins and trap all retinal Schiff bases in their protonated form. Samples were then solubilized in 1% dodecyl-β- D -maltoside (Glycon Biochemicals) for 30 min and centrifuged at 16,000× g for 10 min, and the absorbance of the supernatant was measured. As a standard, detergent-solubilized purified rhodopsin (0.5, 1, 2 and 4 μM) was acid denatured and the absorbance subsequently measured. A plot of the protonated Schiff base absorbance at 440 nm versus rhodopsin concentration yielded an extinction coefficient of 0.0361 μM −1 cm −1 , and this value was used to convert absorbance values at 440 nm to protonated Schiff base concentration. Acid denaturation was also used to follow Meta II decay in concentrated ROS samples. A single sample of RhoP, with or without arrestin, was incubated at 37 °C while gently shaking. Rhodopsin was photoactivated using a 150-W fibre optic light source (>495 nm) for 1 min. Aliquots (10 μl) were removed at given time points, and 20 mM t -bHA was added. The sample was incubated at room temperature for 90 s, after which the sample was diluted 1:10 with 1% dodecyl-β- D -maltoside in acidified buffer (pH <2). For a baseline control, 20 mM hydroxylamine was added to one aliquot, and after 10 min, the sample was solubilized in buffer as described above. The samples were centrifuged at 16,000× g for 10 min before measurement of absorbance. As each aliquot was collected and processed manually at variable temperature, a large margin of error is assumed with respect to time. However, this inaccuracy does not affect the experimental interpretation. Data points were fit to the exponential decay equation y = y 0 + a * e − b * x within the programme Sigma Plot 10.0 (Systat Software). Rhodopsin regeneration assay Time-based regeneration of rhodopsin following the addition of 11- cis -retinal to OpsP was monitored using a Varian Cary 50 spectrophotometer and its associated kinetic scanning programme. Samples were measured in a small-window cuvette (80 μl, 1 cm path length) placed within a temperature-controlled cuvette holder utilising a Peltier chip and circulating water bath. Samples of arrestin, OpsP and ATR were always incubated in the dark at least 30 min before measuring. Manual pipetting was used to quickly mix the sample after the addition of 11- cis- retinal, and no significant sedimentation of the membranes was observed over the time course of the experiment. Absorbance values at 500 nm were plotted versus time and fit to the double exponential equation y = a *(1− e − b * x )+ c *(1− e − d * x ) within the programme Sigma Plot 10.0. For quantifying blocked regeneration in OpsP in complex with arrestin and ATR, a fivefold molar excess (20 μM) of 11- cis -retinal was added, and after 10 min at room temperature, regeneration was quenched with 50 mM hydroxylamine. Although regeneration was only ~90% complete after 10 min, longer incubation times were avoided to minimise arrestin dissociation. Rhodopsin concentration was subsequently determined by the loss of 500 nm absorbance after illuminating the sample. Fluorescence spectroscopy Steady-state fluorescence was measured using a SPEX Fluorolog (1680) instrument as previously described [12] . In this study, the fluorophore NBD was excited at 500 nm to avoid the high optical density of ATR at 380 nm, and emission was collected in 'front-face' mode to minimise inner filter effects. For samples containing OpsP and ATR, 20 mM t -bHA was added 2 min before measurements to remove nonspecific retinal Schiff bases, which quench NBD fluorescence. Emission was collected between 520 and 660 nm (2 nm step size, 0.5-s integration per point). Excitation slits were minimised to 0.05 nm, and emission slits were opened to 4 nm. When measuring dark-state rhodopsin, we found that <2% of the sample was photoactivated during spectrum acquisition. Samples were measured in a quartz cuvette (0.3-mm path length, 80 μl sample volume) with temperature regulation. The fluorescence intensity was determined by integrating the area below the emission spectrum using the programme Sigma Plot 10.0. For the time-based measurement of arrestin I72NBD and all- trans -retinol, a large 1-cm path length cuvette with mini-stir bar (750 μl sample volume) was used. Fluorescence was measured continuously (1-s integration per point) at 550 nm for NBD (500 nm excitation) or 520 nm for retinol (350 nm excitation). Mathematical analysis of titration curves Retinoid titration data were used to fit an expression describing a single-binding site, where B max is the maximal amplitude and K d is the dissociation constant. The factor j represents a y intercept, which is necessary to properly fit some experimental data. Retinoid titration data were also used to fit an expression describing two independent binding sites, where the superscripts '1' and '2' refer to the two distinct binding sites. We noted that the ATR titration data (especially that in Fig. 3a , blue) were generally better fit by the two site-binding expression. These fits suggested that a portion of the OpsP population-bound ATR with 10-fold higher affinity ( K d ~2 μM) than the other ( K d ~30–80 μM). Arrestin titration data were used to fit an expression derived from the definition of K d , as described recently by Sommer et al . [12] , where A is the concentration of arrestin, R is the concentration of receptor and AR is the concentration of the arrestin-receptor complex. The factors j and s allowed the basic binding expression to be appropriately scaled to experimental data. The above equation is suitable for titration experiments carried at concentrations near or above the K d and is ideal for determining stoichiometry. Although K d determination is preferentially carried out at concentrations below the K d , our spectroscopic measurement methods necessitated concentrations hundreds of times greater than the reported K d of the arrestin/Meta II-P complex [13] , [14] , [15] . In addition, our experiments were carried out at ~20 °C, where the rate of Meta II decay is fast enough such that a significant portion of Meta II decays before arrestin binding is complete. This effect is especially pronounced when the ratio of arrestin to receptor is stoichiometric and causes a rounding of the titration curve (that is, higher K d estimation). The limited time resolution of the pull-down assay also contributed to an overestimation of the K d [12] . For these reasons we report apparent K d values. The graphing programme SigmaPlot 10.0 was used to fit curves to experimental data using nonlinear regression algorithms. General experimental conditions Isotonic buffer consisted of 50 mM HEPES buffer pH 7, 130 mM NaCl and 1 mM MgCl 2 . All other experiments were performed in 50 mM HEPES buffer pH 7. Unless otherwise indicated, experiments were performed at ambient room temperature (21–23 °C). When titrating retinoid, a single stock of arrestin and OpsP was prepared and aliquoted equally (118 μl). A dilution series of the retinoid was then prepared in ethanol, and 2 μl from each of these dilutions was added to each aliquot of arrestin and OpsP. The concentrations of the retinoid dilution series was verified by absorbance spectroscopy. When titrating salt, identical aliquots of arrestin and receptor were each diluted onefold with buffer containing increasing concentrations of NaCl or MgCl 2 . How to cite this article: Sommer M. E. et al . Distinct loops in arrestin differentially regulate ligand binding within the GPCR opsin. Nat. Commun. 3:995 doi: 10.1038/ncomms2000 (2012).